Uncoupling conformational states from activity in an allosteric enzyme ATP-phosphoribosyltransferase (ATP-PRT) is a hexameric enzyme in conformational equilibrium between an open and seemingly active state and a closed and presumably inhibited form. The structure-function relationship of allosteric regulation in this system is still not fully understood. Here, we develop a screening strategy for modulators of ATP-PRT and identify 3-(2-thienyl)- l- alanine (TIH) as an allosteric activator of this enzyme. Kinetic analysis reveals co-occupancy of the allosteric sites by TIH and l -histidine. Crystallographic and native ion-mobility mass spectrometry data show that the TIH-bound activated form of the enzyme closely resembles the inhibited l -histidine-bound closed conformation, revealing the uncoupling between ATP-PRT open and closed conformations and its functional state. These findings suggest that dynamic processes are responsible for ATP-PRT allosteric regulation and that similar mechanisms might also be found in other enzymes bearing a ferredoxin-like allosteric domain. Allostery is the change in protein activity triggered by binding of a ligand (effector) at a site different from the active site [1] , [2] . Feedback allosteric circuits are a direct, rapid and efficient mechanism of metabolic control. These feedback allosteric circuits contribute to metabolic homeostasis by translating changes in the concentration of metabolites to enzyme activity and ultimately cellular responses [3] . Protein domains with a ferredoxin-like (FL) βαββαβ topology have been widely co-opted throughout evolution for allosteric control. Particular FL domains have evolved to recognize and respond to one -or sometimes more- molecules of very distinct nature, including nucleotides [4] , heavy metals [5] , and various amino acids. Aspartate carbamoyltransferase (an FL domain containing enzyme) is one of such enzymes, where multiple nucleotides inhibit or activate catalysis. Elegant work describing the complex analysis of regulation by multiple effectors (physiologic ligands) has been carried out [6] . Feedback regulation via amino acid binding to FL domains is widespread in enzymes involved in amino acid biosynthetic pathways (Supplementary Fig. 1 ). Examples in the biosynthesis of aromatic amino acids include eukaryotic phenylalanine-4-hydroxylase (PAH; 1.14.16.1), regulated type Iβ 3-deoxy-D- arabino -heptulosonate 7-phosphate synthase (DAH7PS; 2.5.1.54) [7] and the bacterial and plant chorismate mutase/prephenate dehydratase (PDT; 5.4.99.5/4.2.1.51) [8] . In branched amino acids biosynthesis, proteins regulated via FL domains are the bacterial and plant biosynthetic threonine ammonia-lyase (EC 4.2.1.19) [9] and the bacterial acetohydroxyacid synthase isozyme III (AHAS; EC 2.2.1.6) [10] . Other examples are in Thr, Lys, Met and Ile biosynthesis, the bifunctional chloroplastic aspartokinase/homoserine dehydrogenase 2 (AKHSDH2; 2.7.2.4/ 1.1.1.3), and in Ser biosynthesis, D-3-phosphoglycerate dehydrogenase types I and II (PHGDH; 1.1.1.95). The long form of ATP-phosphoribosyltransferase (ATP-PRT; EC 2.4.2.17), the enzyme that catalyses the first committed step of l- histidine ( l- His) biosynthesis, is also feedback inhibited by l- His [11] , [12] (Supplementary Figs. 2 and 3 ) via a FL domain. Many of these FL-regulated enzymes present in pathogenic bacteria, such as the ATP-PRT from Mycobacterium tuberculosis , are essential and have been proposed as attractive targets for antibacterial drug discovery. Protein domain structure databases place the FL domain of ATP-PRT in the same superfamily as the cyclic-di-AMP receptor family, peptidase S54, and the GlnB proteins [13] , [14] . The defining attribute of the GlnB superfamily is that the FL domains arrange in trimers with the β-sheet of each monomer positioned orthogonally to one another [14] . Because of the common FL fold and functional similarity, the regulatory domain of ATP-PRT has also been associated with the aspartate kinase, chorismate mutase and TyrA (ACT) superfamily [15] . The FL domains of GlnB and ACT have no known evolutionary relationships and represent a superfold that has likely emerged by convergence [16] . Our understanding of the mechanisms of amino acid-binding FL domain-mediated allosteric inhibition comes mostly from the few available crystal structures of free vs. inhibited forms. For T. maritima DAH7PS and PHGDH, the available structures show that effector binding triggers domain reorganization leading to occlusion of the active site [17] , [18] . In the case of ATP-PRT, an early study proposed that l -His binding caused a transition from dimer to hexamer [19] . However, more recent data show that both free and inhibited ATP-PRT are hexameric but that the l -His-bound form is more compact due to a slight rotation of the regulatory domains [12] , [15] , [20] . We now understand crystal structures as being the static snapshots of a continuum of conformations sampled by the enzyme. In this light, ATP-PRT can be described to exist in an equilibrium between a relaxed (R) hexamer and a tense (T) compact hexamer, with l -His binding preferentially to the R state and causing the population to shift to the T state [21] , [22] . In an effort to better understand the allosteric regulation mechanism of ATP-PRT, we implemented a Compound Screening in the Presence of an Inhibitor (CoSPI) strategy (Fig. 1 ). CoSPI makes use of a known inhibitor to provide a targeted and detailed discovery of compounds that have an effect on activity of the enzyme as well as in its regulation. In contrast to most screens employed to date, CoSPI identifies molecules that are only active in the presence of a regulator-enzyme complex. This strategy led us to the discovery of 3-(2-Thienyl- l- alanine) (TIH) as a non-essential activator of M. tuberculosis ATP-PRT. Detailed kinetic measurements and structural characterization of ATP-PRT in the presence of TIH and/or l- His allowed us to probe the mechanism of allosteric regulation in ATP-PRT with unexpected results. Activation and inhibition of ATP-PRT leads to the same overall conformational tightening of the hexamer. This decoupling of activity and conformation indicates that allosteric regulation of ATP-PRT, and perhaps other FL domain containing allosteric enzymes, is more complex than the simple open–closed active–inactive model. Fig. 1 Schematic representation of CoSPI method vs conventional screenings. In the Compound Screening in the Presence of an Inhibitor (CoSPI) strategy, complete IC 50 curves are recorded for a known inhibitor in the presence of each of the test compounds. The enzyme is in blue , substrates in yellow , known inhibitor in red and compound to test in green . The top panels show the single points observed in a conventional screening ( red dots are missed hits, blue is an activator and pink an inhibitor). The bottom panels show the information-rich patterns observed using CoSPI. Curves depict simulated data for an inhibitor with IC 50 = 20 µM, Hill number of 1 and capable of full inhibition (100 to 0% activity). The red curve are the data for the known inhibitor in the absence of other molecules. a Effects in the potency of the inhibitor. Green , increase in the apparent affinity of the inhibitor. Orange , decrease in the apparent affinity of the inhibitor. b Effects in the activity of the enzyme independently of the inhibitor. Blue , increase in the activity of the enzyme. Pink , decrease in the activity of the enzyme. c Effects in inhibitor-enzyme cooperativity. Cyan , increase in the cooperativity of inhibition. Grey , decrease in the cooperativity of inhibition Full size image CoSPI identifies TIH as an activator of ATP-PRT We carried out a small, targeted version of CoSPI, to demonstrate its ability to uncover non-canonical regulators of enzyme function. By following the formation of phosphoribosyl-ATP (PR-ATP, ε 290 = 3600 M −1 cm −1 ), we tested the effect of 11 commercially available l -His analogues, at a single concentration (1 mM), on the inhibition of ATP-PRT by l -His (Fig. 2a and Supplementary Fig. 4 ). Using as reference the activity values of uninhibited enzyme and the IC 50 of l -His in the absence of any additional compounds (dashed lines in Fig. 2a ), the selection of the best candidates was straightforward. Analogues 2 and 6 showed a change in l- His IC 50 and uninhibited maximal activity. TIH, compound 2, was chosen for further characterization as it had the greatest effect. Addition of TIH to the reaction mixture resulted in a linear increase in the l- His IC 50 , and a hyperbolic (saturable) increase in the reaction velocity (Fig. 2b, c ). We confirmed the activation of ATP-PRT by TIH by determining the concentration required to half-maximal activation ( AC 50 ) (Fig. 2d ). TIH increases ATP-PRT activity up to 433 ± 18 %, with an AC 50 of 1.5 ± 0.2 mM. Fig. 2 CoSPI discovery of a non-essential activator of ATP-PRT. a l- His IC 50 and %Activity data obtained in the presence of each of 11 l- His analogues using CoSPI. The dashed lines mark l- His IC 50 and the activity of uninhibited ATP-PRT. Error bars indicate the s.d. Number of replicates ( n ) = 3 b Representative inhibition curves determined for l- His in the presence of 0 ( black ), 0.5 ( purple ), 1 ( orange ), 2 ( yellow ) and 4 ( green ) mM compound 2, TIH (shown in the upper right corner ). Circles are experimental measurements and lines the best fit to Eq. 2 in Methods section. c Replot of the data in b , showing hyperbolic increase in ATP-PRT activity ( circles ) and linear increase in l- His IC 50 ( squares ), in the presence of TIH. The lines are the best fit to Eq. 1 in Methods and a linear regression of the data, respectively. Error bars indicate the s.e.m. d Steady-state kinetics of ATP-PRT activation by TIH. Circles are data points and the line is the best fit to Eq. 3 in Methods section, n = 2. e General modifier mechanism depicting an activator, E, enzyme; S, substrate; A, activator; P, product. f Double-reciprocal plot highlighting the non-essential activation pattern obtained when varying the concentration of TIH. Circles are data points obtained with 0 ( black ), 0.25 ( red ), 0.8 ( blue ) and 4 ( green ) mM TIH and lines are the best fit of the entire data set to Eq. 4 in Methods section. Error bars indicate the s.d., n = 2 Full size image TIH increases ATP-PRT turnover rate According to the Botts and Morales general modifier mechanism (Fig. 2e ) [23] , [24] , the presence of a modifier (either an inhibitor or an activator) might have an effect on the dissociation constant of the ternary enzyme-substrate-modifier complex, this effect is given by the constant α. In addition, the modifier can have an effect on k cat , which is described by the coefficient β. Non-essential activation is generally characterized by a ligand that can bind and activate an enzyme, not being essential for enzymatic activity. Values of α lower than 1 and values of β higher than 1 are usually observed. However, mixed-type systems where α and β are higher than 1 are also possible, as are systems where α and β are both lower than 1 [25] . We performed measurements of ATP-PRT activation by TIH at different concentrations of either of the substrates, ATP or PRPP. Coefficients α and β were consistent with non-essential activation in both cases (Fig. 2f , Supplementary Figs. 5 and 6 ). For ATP we obtained a K A,ATP value of 1.5 ± 0.2 mM, an α ATP of 1.4 ± 0.2 and a β ATP value of 4.9 ± 0.2. The activity of the unactivated reaction was 0.17 ± 0.01 s −1 and the K m,ATP 0.10 ± 0.01 mM, in close agreement with values previously reported [12] . In the case of varying concentrations of PRPP, K A,PRPP was 2.1 ± 0.6 mM, α was 1.1 ± 0.4 and a β 4.9 ± 0.5. The activity of the unactivated reaction was 0.21 ± 0.01 s −1 and the K m,PRPP 0.19 ± 0.03 mM. These results indicate that TIH has little effect on the stability of the tertiary complex, but is able to increase the catalytic rate by up to 490%. l -His and TIH binding are mutually affected We performed single inhibition measurements with co-variation of either substrate, ATP or PRPP, and l -His. Results showed linear uncompetitive inhibition by l -His vs. ATP, with a K i,ATP of 20 ± 1.0 µM, and linear noncompetitive inhibition vs. PRPP, with a K i,PRPP of 16 ± 1.0 µM as previously reported [12] . Following the method described by Andi and collaborators [26] , we repeated the inhibition experiment at four different concentrations of TIH (0, 0.25, 0.8 and 4 mM) (Fig. 3a ). 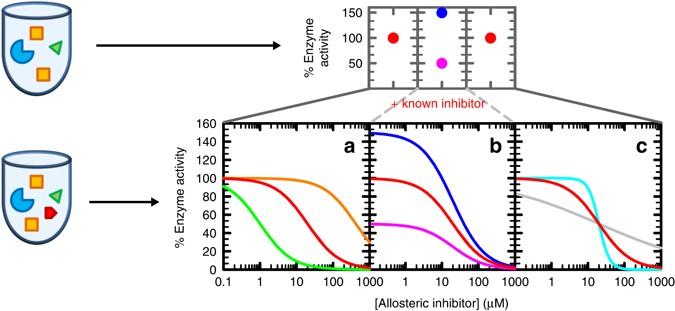Fig. 1 Schematic representation of CoSPI method vs conventional screenings. In the Compound Screening in the Presence of an Inhibitor (CoSPI) strategy, completeIC50curves are recorded for a known inhibitor in the presence of each of the test compounds. The enzyme is inblue, substrates inyellow, known inhibitor inredand compound to test ingreen. Thetoppanels show the single points observed in a conventional screening (red dotsare missed hits,blueis an activator andpinkan inhibitor). Thebottompanels show the information-rich patterns observed using CoSPI. Curves depict simulated data for an inhibitor withIC50= 20 µM, Hill number of 1 and capable of full inhibition (100 to 0% activity). The red curve are the data for the known inhibitor in the absence of other molecules.aEffects in the potency of the inhibitor.Green, increase in the apparent affinity of the inhibitor.Orange, decrease in the apparent affinity of the inhibitor.bEffects in the activity of the enzyme independently of the inhibitor.Blue, increase in the activity of the enzyme.Pink, decrease in the activity of the enzyme.cEffects in inhibitor-enzyme cooperativity.Cyan, increase in the cooperativity of inhibition.Grey, decrease in the cooperativity of inhibition Increasing the concentration of TIH resulted in higher values of V max and, therefore k cat, and K i,ATP for l -His inhibition (Table 1 ). As expected, the affinity of ATP was not considerably affected. A secondary replot of the data in Fig. 3a revealed a linear dependence of both the slopes and the intercepts as a function of l -His concentration (Fig. 3b ). Tertiary replots of the slopes and intercepts of the data in Fig. 3b showed an exponential dependence on activator concentration (Fig. 3c ). Three different K A values could be determined from the tertiary replots using eq. 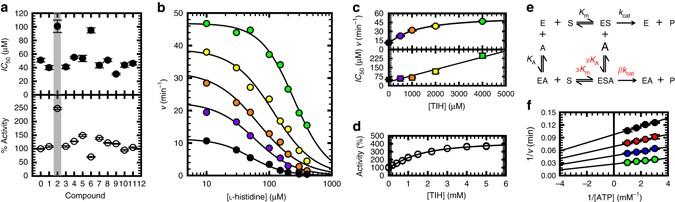Fig. 2 CoSPI discovery of a non-essential activator of ATP-PRT.al-HisIC50and %Activity data obtained in the presence of each of 11l-His analogues using CoSPI. The dashed lines markl-HisIC50and the activity of uninhibited ATP-PRT.Error barsindicate the s.d. Number of replicates (n) = 3bRepresentative inhibition curves determined forl-His in the presence of 0 (black), 0.5 (purple), 1 (orange), 2 (yellow) and 4 (green) mM compound 2, TIH (shown in theupper right corner).Circlesare experimental measurements andlinesthe best fit to Eq.2in Methods section.cReplot of the data inb, showing hyperbolic increase in ATP-PRT activity (circles) and linear increase inl-HisIC50(squares), in the presence of TIH. Thelinesare the best fit to Eq.1in Methods and a linear regression of the data, respectively.Error barsindicate the s.e.m.dSteady-state kinetics of ATP-PRT activation by TIH.Circlesare data points and thelineis the best fit to Eq.3in Methods section,n= 2.eGeneral modifier mechanism depicting an activator, E, enzyme; S, substrate; A, activator; P, product.fDouble-reciprocal plot highlighting the non-essential activation pattern obtained when varying the concentration of TIH.Circlesare data points obtained with 0 (black), 0.25 (red), 0.8 (blue) and 4 (green) mM TIH andlinesare the best fit of the entire data set to Eq.4in Methods section.Error barsindicate the s.d.,n= 2 7 (Methods; Table 2 ). Each of the K A values corresponds to the affinity of TIH to one of the following complexes, ES P (intercept of the slope, K A1,ATP ), ES P S A (intercept of the intercept, K A3,ATP ) and ES P S A I (slope of the intercept, K A4,ATP ), where I is the inhibitor, S A is ATP and S P is PRPP, as illustrated in the model (Fig. 3d ). The ratio of K A3,ATP / K A4,ATP reports on the affinity of the activator for the ES A S P complex, in the presence of the inhibitor, and is characterized by α 3/4,ATP = 2.60 ± 0.66; the value higher than 1 indicates that TIH has higher affinity for ATP-PRT in complex with l -His. Also determined from the tertiary replots (Supplementary Fig. 8a and Supplementary methods ), the activation of ATP-PRT by TIH is higher when TIH binds to ATP-PRT in the presence of l- His. An 18-fold activation by TIH was observed in the presence of both substrates and l -His in contrast to a 6-fold activation in the absence of inhibitor; when TIH binds to ATP-PRT in complex with PRPP only a 11-fold activation is observed (Table 2 and Fig. 3d ). When varying PRPP concentration (Supplementary Figs. 7 and 8b ), four different K A ’s could be determined. Once again, the results show that TIH has higher affinity for ATP-PRT in complex with l- His with values of α 1/2,PRPP = 1.92 ± 0.33 and α 3/4,PRPP = 3.27 ± 0.98, and fold-activation values were as high as 29, in the presence of l- His and ATP. Fig. 3 l- His inhibition kinetics in the presence of TIH. a Four double-reciprocal plots showing linear uncompetitive inhibition patterns determined for l- His in the presence of 0 ( black ), 0.25 ( red ), 0.8 ( blue ) and 4 ( green ) mM TIH, at fixed variable concentrations of ATP. Results are representative of two independent experiments. Points are experimental data obtained with 0 ( black circles ), 12 ( white circles ), 24 ( black squares ) and 36 (white squares) µM l- His. Lines are the best fit of each uncompetitive pattern data set to Eq. 5 in Methods section. b Secondary replot of the slopes ( circles ) and intercepts ( squares ) of the data shown in a . c Tertiary replots of the slopes ( top panel ) and intercepts ( lower panel ) of the data shown in b . Slope of the intercept ( triangles ), intercept of the intercept ( diamond s) and intercept of the slope ( hexagons ). Lines are the best fit to Eq. 7 in Methods section. d Kinetic model for a combination of uncompetitive inhibition and non-essential activation. The complexes in boxes are in equilibrium. The blue box indicates that this complex is always present in the assay. E, Enzyme; S A , ATP; S P , PRPP; A, TIH; I, l- His; P, Product Full size image Table 1 Steady-state kinetic parameters for ATP-PRT inhibition in the presence of TIH Full size table Table 2 Steady-state kinetic parameters for ATP-PRT activation in the presence of l- His Full size table TIH rescues ATP-PRT activity in the presence of l- His At a saturating concentration of l -His (400 µM, 20-fold K i ), ATP-PRT is fully inhibited, showing no activity (Fig. 4a ). Recovery of the activity can be achieved simply by addition of TIH to the inhibited reaction mixture. At a concentration close to 4 mM TIH (2-fold higher than K A ~ 2 mM) 100% of the activity is restored and further activation is achieved with higher concentrations of TIH. Figure 4b shows a contour map that better illustrates the entire activity landscape obtained for ATP-PRT, in the presence of l- His and TIH, at all concentrations tested. 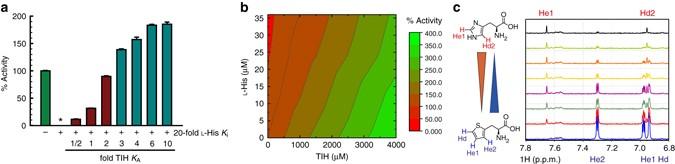Fig. 4 Competition between TIH andl-His.aATP-PRT activity in the absence ofl-His (green bar), in the presence of anl-His concentration equivalent to 20-foldKi(0.4 mM;star) and in the presence of 0.4 mMl-His plus increasing concentrations of TIH (dark redandcyan bars,KA= 2 mM).Error barsindicate the s.d.,n= 3.bContour plot of ATP-PRT activity landscape in the presence of bothl-His and TIH.cSTD-NMR of TIH andl-His with 20 μM ATP-PRT. TIH concentration was kept at 400 μM, while the concentration ofl-His was varied, 0, 50, 100, 150, 400, 800, 1600 and 3000 μM, from theblue bottomtrace, to theblack toptrace. Experiments were performed in 50 mM sodium phosphate buffer at pH 8.0.Redand navy bluetriangles indicate ATP-PRT occupancy byl-His and TIH, respectively Simultaneous binding of TIH and l- His to the hexamer was confirmed through a competition saturation transfer difference (STD) NMR experiment [27] . In an STD NMR experiment, signals are observed only for ligand protons in contact with the protein. In the absence of l- His signals of the TIH protons are observed (Fig. 4c , bottom spectrum). Increasing concentrations of l- His result in the progressive reduction of the TIH peaks and the appearance of l- His proton signals, indicating displacement of TIH by l- His. Fig. 4 Competition between TIH and l- His. a ATP-PRT activity in the absence of l- His ( green bar ), in the presence of an l- His concentration equivalent to 20-fold K i (0.4 mM; star ) and in the presence of 0.4 mM l- His plus increasing concentrations of TIH ( dark red and cyan bars , K A = 2 mM). Error bars indicate the s.d., n = 3. b Contour plot of ATP-PRT activity landscape in the presence of both l- His and TIH. c STD-NMR of TIH and l- His with 20 μM ATP-PRT. TIH concentration was kept at 400 μM, while the concentration of l- His was varied, 0, 50, 100, 150, 400, 800, 1600 and 3000 μM, from the blue bottom trace, to the black top trace. Experiments were performed in 50 mM sodium phosphate buffer at pH 8.0. 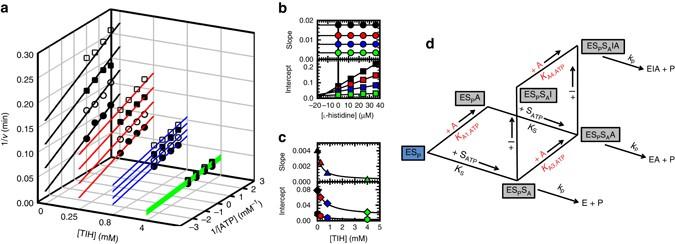Red and n avy blue triangles indicate ATP-PRT occupancy by l- His and TIH, respectively Full size image Both TIH and l -His-bound ATP-PRT are in the T conformation We solved the crystal structures of ATP-PRT in complex with TIH or l -His by molecular replacement using the unliganded coordinates of the ATP-PRT ternary complex with l -His and AMP (1NH8) as a search model. Fig. 3 l-His inhibition kinetics in the presence of TIH.aFour double-reciprocal plots showing linear uncompetitive inhibition patterns determined forl-His in the presence of 0 (black), 0.25 (red), 0.8 (blue) and 4 (green) mM TIH, at fixed variable concentrations of ATP. Results are representative of two independent experiments. Points are experimental data obtained with 0 (black circles), 12 (white circles), 24 (black squares) and 36 (white squares) µMl-His.Linesare the best fit of each uncompetitive pattern data set to Eq.5in Methods section.bSecondary replot of the slopes (circles) and intercepts (squares) of the data shown ina.cTertiary replots of the slopes (top panel) and intercepts (lower panel) of the data shown inb. Slope of the intercept (triangles), intercept of the intercept (diamonds) and intercept of the slope (hexagons).Linesare the best fit to Eq.7in Methods section.dKinetic model for a combination of uncompetitive inhibition and non-essential activation. The complexes inboxesare in equilibrium. Theblue boxindicates that this complex is always present in the assay. E, Enzyme; SA, ATP; SP, PRPP; A, TIH; I,l-His; P, Product Crystals of the two complexes grew in identical crystallization conditions and to comparable resolution, thus being an ideal case for a direct and detailed comparison between structures (Table 3 ). All ATP-PRT crystals obtained in complex with either l -His or TIH invariably belonged to the H 3 2 space group with one protein molecule in the asymmetric unit. The hexamer representing the biological assembly of ATP-PRT was obtained by symmetry operations preventing us from solving the structure of an ATP-PRT complex with both l -His and TIH. Table 3 Data collection and refinement statistics (molecular replacement) Full size table As expected on the basis of the overall structural similarity between the two ligands and the results of the competition kinetics experiments, TIH was found to bind in the same allosteric site as l -His (Fig. 5a, d and g ), a site defined by opposite and complementing surfaces of two adjacent regulatory FL-like domains. The position of the ligand in each complex was inferred by the presence of positive density in the unbiased difference map derived by molecular replacement (Supplementary Fig. 9 ). Fitting of the ligands and refinement of the structure resulted in identical ligand orientation (Fig. 5d and g ). We confirmed the identity of TIH by calculating the anomalous scattering difference map for a data set of the complex collected at 1.8 Å, which exhibited positive density for the sulphur in the thiophenyl moiety and allowed unambiguous assignment of the correct orientation of the ring (Supplementary Fig. 10a ). Side chains of the residues directly interacting with the ligand assume identical conformations in the two complexes with the only exception of D216 (Fig. 6a and b ). In the ATP-PRT/ l- His complex D216 interacts with the l -His side chain via a water molecule-mediated H-bond to ND1, but in the complex with TIH the water molecule is missing and its position occupied by one of two observed conformations for the D216 side chain which is oriented towards the thiophenyl ring. Taken together, the overall similarity between “inhibited” and “activated” structures and the differential conformation of D216 in both complexes could indicate that D216 is a “trigger” for inhibition of ATP-PRT. Steady-state kinetics studies on the D216V mutant support the interpretation of a specific role for D216 in l -His recognition and inhibition. D216V ATP-PRT is no longer inhibited by l -His (up to 10 mM); however, it is still activated by TIH, in the presence or absence of l -His, with similar affinity to the wild type (Fig. 6c and d ). The other noticeable structural difference in the allosteric binding site is the absence in the TIH complex of the H-bond observed between HE2 of l -His and the carbonyl oxygen of A273. The missing H-bonds are likely to account for the three orders of magnitude difference in the apparent affinity of the two ligands and their opposite effect on enzymatic activity (Fig. 6 ). Fig. 5 Crystal structure and native IM-MS of apo-, l- His-bound and TIH-bound ATP-PRT. Cartoon representation of the allosteric binding site in the hexamer, surface representation viewed from the top and native drift time distribution of: a , b , c Apo- (PDB code 1NH7); d , e , f l- His-bound (PDB code 5LHU), and g , h , i TIH-bound (PDB code 5LHT) ATP-PRT. Allosteric domains are coloured in yellow while the catalytic domains are coloured in blue . The bars represent the span of the different molecule complexes. Distances have been measured between coupled Cα atoms of I269 ( yellow bars ) and I129 ( blue bars ). The black arrow on c indicates the fraction of unliganded ATP-PRT in the T-state Full size image Fig. 6 Differential conformations and kinetics of wild-type and D216 ATP-PRT in the presence of l- His or TIH. Cartoon representation highlighting the H-bonds surrounding l- His a and TIH b in their respective crystal structures. The D216 side chain in the TIH-bound ATP-PRT structure could be fitted in two conformations with 0.35 and 0.65 occupancy. Steady-state kinetics of ATP-PRT inhibition by l- His c , and activation by TIH d . WT ( black circles) , D216 V ( red circles ) and D216 V + 2 mM l- His ( blue circles ), error bars indicate the s.d., n = 3. Circles are experimental measurements and lines are the best fit to Eq. 2 (Methods section) for inhibition by l- His and Eq. 4 (Methods section) for activation by TIH. Data for D216 V inhibition by l- His were fit to a linear regression. For WT, an IC 50 for l- His of 22 ± 4 μM and an AC 50 for TIH of 1.5 ± 0.2 mM were obtained. For D216 V, an AC 50 for TIH of 1.7 ± 0.1 mM was obtained, which did not change in the presence of 2 mM l- His, with an AC 50 of 1.5 ± 0.1 mM. l- His (up to 10 mM) did not change D216 V activity and therefore an IC 50 could not be determined Full size image The comparison between the structures of both the monomer and the crystallographic hexamer revealed that the l -His inhibited and the TIH activated complexes are highly superimposable and share the same tense (T) conformation so far attributed to the inactive state of the enzyme (Supplementary Fig. 11 ) [19] , [20] , [28] . Furthermore, no appreciable differences between the two complexes were observed in the side-chain orientation of the residues expected to be involved in substrate and/or product binding by virtue of similarity with the E. coli ATP-PRT in complex with PR-ATP (PDB code: 1Q1K) [28] and C. jejuni ATP-PRT in complex with ATP (PDB code: 4YB7) [20] (Supplementary Fig. 12 ). The mean global RMSD between the two complexes calculated over the entire sequence (residues 1–284) was 0.12 and 0.61 Å for the backbone and heavy atoms, respectively. The RMSD value between the open unliganded ATP-PRT (1NH7) and the structures in this work was of 4.24/4.56 Å (backbone/heavy atoms) and 4.24/4.55 Å for the l -His- and TIH-complexes, respectively. The crystallographic structures at 1.8 Å of the ATP-PRT/TIH complex obtained from different crystallization conditions consistently showed the hexamer in a T-state (Supplementary Fig. 10b ). Native mass spectrometry supports R to T conformation shift To complement our crystallographic results we employed native ion-mobility mass spectrometry (IM-MS) to investigate the equilibrium between the R- and T-states in the presence of either l -His or TIH. We obtained data for unligated ATP-PRT and in complex with l -His or TIH, at neutral pH (6.8) and in mildly alkaline pH (9.0) conditions in which ATP-PRT is more active [12] (Supplementary Table 1 ). Results at neutral pH (Fig. 5 ) showed the existence of a pre-existing equilibrium between the R- (drift time of 51.2 ms) and T- (drift time of 44.0 ms) states, with a strong preference for the R-state. Addition of either l -His or TIH shifted the equilibrium towards shorter drift times (44.1 and 44.2 ms, respectively), characteristic of the T-state. At basic pH, unligated, l -His and TIH-bound ATP-PRT are all in the T-state (Supplementary Fig. 13 ). Target-based small-molecule screenings are a valuable and widely used approach for lead generation in drug discovery. In traditional screenings compounds are tested against purified enzymes, with the goal of detecting enzyme inhibition [29] , [30] , activation [31] , or binding to the target protein [32] , while other screenings test for secondary ligands that only bind after the first ligand binds [33] , [34] . Despite their undisputed usefulness, traditional screens fail to detect compounds displaying less common or peculiar effects, such as influencing the efficacy or affinity of a known effector, or altering effector–enzyme cooperativity. In order to screen for these effects, we developed CoSPI, a targeted screen of small molecules. The screen is carried out in the presence of a known inhibitor, and consists of determining and evaluating the entire inhibition profile ( IC 50 curve) of the known inhibitor in the presence of a single fixed concentration of each of the compounds. Hill number ( n H ), V max and IC 50 are then estimated from such curves and compared. Three limiting behaviours can potentially be observed using a CoSPI design (Fig. 1 ). First, compounds that have no effect on their own but are able to increase or decrease the potency of the known inhibitor (Fig. 1a ). Second, compounds able to alter the enzyme activity independently of the known inhibitor (Fig. 1b ). And third, compounds that do not alter enzyme activity but alter the inhibitor-enzyme cooperativity (Fig. 1c ). As proof of concept, we used the CoSPI strategy to screen 11 l- His analogues for their ability to modify M. tuberculosis ATP-PRT activity in the presence of its allosteric inhibitor l- His. The outcome of the screen was simple and clear (Fig. 2a ), and lead to the discovery of TIH, the first reported allosteric activator of ATP-PRT and in the whole histidine biosynthesis pathway. Allosteric activators have only recently emerged as valuable tools for the study of conformational changes associated with enzyme activation, and of the biological consequences of enzyme activation in the context of a specific signalling/metabolic pathway [35] . TIH is a non-essential ATP-PRT activator of weak molar potency with K A,ATP value of 1.5 ± 0.2 mM and K A,PRPP value of 2.1 ± 0.6 mM. Nonetheless, it is able to activate ATP-PRT by up to 500%. TIH activation originates solely from a V -type effect, this is, it increases the catalytic rate (β-value of 4.9) but has no effect on K m (α-value ~1); this is a different type of activation from most cases reported to date [36] , [37] , [38] , [39] . To the best of our knowledge, a fivefold increase in k cat is one of the highest increases reported for a small-molecule allosteric activator. Having a similar structure and judging by its effect on l- His IC 50 (Fig. 2b and c ) it was expected that TIH and L -His bound at the same site. The results of the inhibition studies with co-variation of either of the substrates and L -His, at four different concentrations of TIH (Fig. 3a and Supplementary Fig. 7a ) further supported this idea. In these experiments, increasing concentrations of TIH did not significantly affect the affinity of the substrates, but K i values for L -His increased linearly, indicating a strong effect of TIH on l- His potency (Table 1 and Supplementary Fig. 7b ). Furthermore, and despite its weak potency, TIH at a concentration of twice K A (4 mM) was sufficient to fully activate ATP-PRT in the presence of l- His at a concentration ≈ twice K i (36 μM). Under these conditions V max reached values close to those obtained in the presence of saturating concentration of TIH (absence of l- His), V a,max , justifying the increase in fold-activation values from 6 to 18-fold. To confirm this behaviour, ATP-PRT activity was tested at increasing concentrations of TIH in the presence of l- His at a concentration of 20 times K i (Fig. 4a ), which fully abolishes activity. Again we saw that TIH at a concentration of 2 times K A is sufficient to rescue ATP-PRT to normal activity levels. This apparently counterintuitive behaviour, indicative of a “kinetic superiority” of a low affinity ligand over a high affinity ligand may occur because there are six l- His binding sites in the ATP-PRT hexamer [12] , [19] . The n H for l- His inhibition is 1.5 12 , suggesting that occupation of four of the six binding sites is sufficient for full inhibition of the hexamer, leaving two sites available for TIH to bind and activate ATP-PRT (Supplementary Fig. 14 ). In agreement with this hypothesis, TIH affinity is higher when l- His is bound to ATP-PRT, as revealed by values of α 3/4,ATP , α 1/2,PRPP and α 3/4,PRPP of 1.9-, and 3.3- and 2.6-fold, respectively. This preference of TIH for the ATP-PRT- l- His complex is substrate independent. In addition, the fold-activation obtained in the presence of l- His is considerably higher than the fold-activation obtained in its absence (Table 2 and Supplementary Fig. 7e ), this is because the very low V max values observed in the presence of l- His increase substantially upon addition of TIH, until reaching V a,max , giving higher values of fold-activation. There have been a few reports of activators of bacterial enzymes in the literature, including activators of cylindrical proteases [40] , [41] , proteasome-related HslV peptidase [42] and glycoside hydrolase [39] . Nonetheless, TIH seems to be a distinct small-molecule activator of a bacterial enzyme, binding in the same site as the natural allosteric inhibitor. The similarity between the crystallographic structures of the ATP-PRT hexamer in complex with the l- His or with TIH was surprising. Despite exerting an opposite effect on the enzymatic activity, both induce a rigid body conformational change that re-orients the regulatory domain with respect to the catalytic region leading to the compaction of the hexamer characteristic of the T-state. To rule out the possibility that this was a crystallization artefact, we performed measurements in the “vapour phase” using native IM-MS, with equivalent results. Our data suggest that there is not direct correlation between R- and T-states and active and inactive conformations in ATP-PRT. Instead, it is likely that other conformational states, less populated than R- and T-, are critical for activity and/or that there is an important dynamic contribution to the allosteric mechanism. Given that substrate binding and product release can only take place in the R state, the R- and T-states might reflect the functional catalytic ‘cycle’ of ATP-PRT. We hypothesize that activators and inhibitors have opposite effects on the rate of sampling of the conformational ensemble. Thus, an activator may increase turnover by accelerating the sampling rate, while an inhibitor might slow it down. This hypothesis is consistent with the fact that TIH activation is solely due to an increase in V max . A detailed characterization of the conformational equilibrium exchange rates in the presence and absence of effectors will be required to test this hypothesis and is currently in progress. 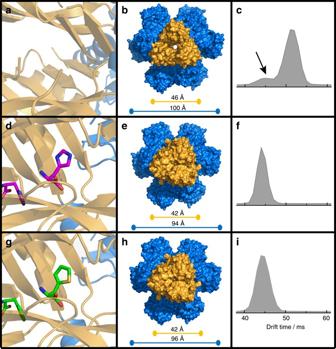Fig. 5 Crystal structure and native IM-MS of apo-,l-His-bound and TIH-bound ATP-PRT. Cartoon representation of the allosteric binding site in the hexamer, surface representation viewed from the top and native drift time distribution of:a,b,cApo- (PDB code 1NH7);d,e,fl-His-bound (PDB code 5LHU), andg,h,iTIH-bound (PDB code 5LHT) ATP-PRT. Allosteric domains are coloured inyellowwhile the catalytic domains are coloured inblue. Thebarsrepresent the span of the different molecule complexes. Distances have been measured between coupled Cα atoms of I269 (yellow bars) and I129 (blue bars). Theblack arrowoncindicates the fraction of unliganded ATP-PRT in the T-state 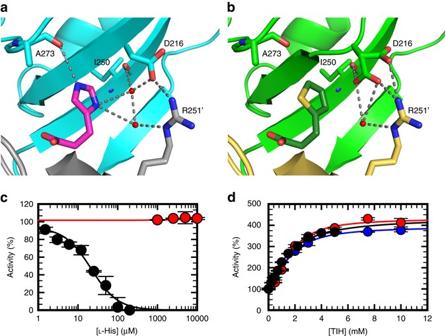Fig. 6 Differential conformations and kinetics of wild-type and D216 ATP-PRT in the presence ofl-His or TIH. Cartoon representation highlighting the H-bonds surroundingl-Hisaand TIHbin their respective crystal structures. The D216 side chain in the TIH-bound ATP-PRT structure could be fitted in two conformations with 0.35 and 0.65 occupancy. Steady-state kinetics of ATP-PRT inhibition byl-Hisc, and activation by TIHd. WT (black circles), D216 V (red circles) and D216 V + 2 mMl-His (blue circles),error barsindicate the s.d., n = 3.Circlesare experimental measurements andlinesare the best fit to Eq.2(Methods section) for inhibition byl-His and Eq.4(Methods section) for activation by TIH. Data for D216 V inhibition byl-His were fit to a linear regression. For WT, anIC50forl-His of 22 ± 4 μM and anAC50for TIH of 1.5 ± 0.2 mM were obtained. For D216 V, anAC50for TIH of 1.7 ± 0.1 mM was obtained, which did not change in the presence of 2 mMl-His, with anAC50of 1.5 ± 0.1 mM.l-His (up to 10 mM) did not change D216 V activity and therefore anIC50could not be determined Of particular interest is the possibility that the uncoupling between R- and T-states and activity observed for ATP-PRT might be a feature of other ferredoxin-like domain-containing allosteric enzymes. Materials Buffers and l- His were purchased from Fisher Scientific. Except if specified otherwise, all other chemicals were purchased from Sigma-Aldrich. Ni-NTA resin and BL21(DE3)pLysS cells were purchased from Millipore. Complete EDTA-Free protease inhibitor was purchased from Roche. Protein purification All steps of ATP-PRT and PPase purification were performed at 4 ˚C using an AKTA purifier 10 (GE Healthcare). Frozen BL21(DE3)pLysS ( pJ411::hisG and pJ411::ppa ) 50 grams of cells were thawed on ice, resuspended in buffer A (20 mM triethanolamine (TEA) pH 7.8, 300 mM NaCl, and 50 mM imidazole containing lysozyme, Complete® protease inhibitor cocktail and DNase) and lysed by sonication. After centrifugation at 25000 g for 30 min, the soluble fraction was loaded on a 100 ml Ni-NTA column and protein eluted by a 0 to 100% gradient of buffer B (20 mM TEA pH 7.8, 300 mM NaCl and 500 mM imidazole). UV-Vis peak fractions were analysed by SDS-PAGE, performed on a PhastSystem (GE Healthcare). Fractions containing only ATP-PRT or PPase were pooled, dialyzed into 20 mM TEA (pH 7.8), concentrated, flash-frozen and stored at −80 ˚C. This protocol allowed the purification to homogeneity of 1 g of ATP-PRT and 0.5 g of PPase. ATP-PRT concentration was determined using absorbance at 280 nm ( ε 280 = 20,800 M −1 cm −1 ). After the Ni-NTA column step, ATP-PRT protein for crystallization was further purified by gel filtration using a Sephadex S200 16/600 column and concentrated in the elution buffer (20 mM Tris-HCl pH 7.8, 100 mM NaCl) to a final concentration of 13 mg/ml before flash freezing. ATP-PRT activity measurements Steady-state kinetic measurements were conducted at 25 °C ± 0.2 °C with a Shimadzu UV-2550 spectrophotometer equipped with dual-beam optics and a Peltier system for temperature control. Initial velocities for the forward reaction of ATP-PRT were measured by following the formation of PR-ATP ( ε 290 = 3,600 M −1 cm −1 ), in the presence of PPase. Pyrophosphatase is essential for this assay, as the equilibrium constant lies towards formation of ATP and PRPP. A typical reaction mixture contained 50 mM Tris-HCl (pH 8.5), 7 mM MgCl 2 , 200 mM KCl, 3 mM ATP, 1.5 mM PRPP, 600 nM PPase and 450 nM ATP-PRT. l- His analogue screening To determine the effect of 11 commercially available analogues on l- His, ATP-PRT activity was assayed in the presence of saturating concentrations of substrates and metals, variable concentrations of l- His and in the presence of 1 mM of each of the analogues (with the exception of compound 1, where a concentration of 0.9 mM was used). To determine the effect of each analogue on enzyme activity (in the absence of l- His), ATP-PRT activity was measured in the presence of saturating concentrations of substrates and metals, and variable concentrations of each analogue (up to 5 mM). Activation kinetics To determine the steady-state activation parameters and patterns associated with TIH, ATP-PRT activity was studied in the presence of variable concentrations of one substrate, PRPP or ATP, fixed saturating concentrations of the co-substrate (ATP or PRPP) and metals, and several fixed concentrations of TIH. Inhibition kinetics in the presence of activator To determine the interaction between l- His and TIH, ATP-PRT activity was studied in the presence of variable concentrations of one substrate, PRPP or ATP, fixed saturating concentrations of the other substrate (ATP or PRPP) and metals, and several fixed concentrations of l- His. The experiment was repeated at several fixed concentrations of TIH. Activity rescue by TIH ATP-PRT activity was studied in the presence of 0.4 mM l- His, a concentration 20-fold higher than l- His K i , which fully inhibited ATP-PRT. Increasing concentrations of TIH were then added to the reaction, up to 8 mM TIH, a concentration 4-fold higher than TIH K A . 1 H NMR spectroscopy NMR spectra were recorded at 25 °C on a Bruker Avance-600 spectrometer equipped with a triple resonance cryo-probe and operating at a 1 H frequency of 600 MHz. Saturation transfer difference (STD) spectra [43] of 20 µM ATP-PRT in the presence of fixed concentration of TIH and variable concentrations of l- His were recorded in 50 mM sodium phosphate buffer (pH 8.0). Spectra with on-resonance pre-saturation of the enzyme at 0.8 ppm were recorded with a saturation time of 2 s. An off-resonance control spectrum was recorded with a saturation time of 2 s. Water suppression was achieved by excitation sculpting [44] . Data processing and spectral subtractions were performed using Bruker TopSpin 3.2 software. Crystallization and X-ray data collection All crystals of ATP-PRT complexes with either l- His or TIH were obtained by co-crystallization experiments at 18 °C using the sitting drop vapour diffusion method. Drops of 0.2 µl (protein stock:well solution 1:1) were set-up with the assistance of the Oryx protein crystallization robot. Protein concentration was 9.3 mg/ml whereas the ligands concentration was 100 µM and 5.5 mM for l- His and TIH, respectively. Crystals of ATP-PRT complexes with TIH and l- His were obtained from condition 4 of Classics Lite Suite crystallization screen by Qiagen (2.5 %(v/v) isopropanol, 1.0 M ammonium sulphate). Crystals of ATP-PRT in complex with TIH grown in the presence of ATP, although no positive density for ATP molecule could be located, were obtained from condition 71 of the Protein Complex Suite by Qiagen (0.1 M Sodium acetate anhydrous pH 5.0, 1.5 M Ammonium sulphate). Crystals were frozen adding 20 % (v/v) glycerol to the mother liquor for cryo-protection and stored in liquid nitrogen until data collection. Diffraction data were collected at beamline IO4 at the Diamond Light Source, UK. Data collection temperature was 100 K. Wavelength for both ATP-PRT/TIH and ATP/PRT/ l- His datasets was 0.9282. Integration and scaling were performed using XDS and XSCALE via xia2 expert system for X-ray diffraction data processing [45] , [46] . Crystals belong to the rhombohedral space group H 3 2 with one molecule in the crystallographic asymmetric unit, which gives a solvent content of 54–56%. Subsequent data handling was carried out using the CCP4 software package [47] . Structure determination and refinement Molecular replacement was carried out with PHASER [42] , using as a search model the coordinates of M. tuberculosis ATP-PRT complexed with l- His and AMP (PDB code 1NH8), but with the ligands and solvent molecules removed. Models were improved and refined alternating cycles of model correction by Coot [43] and restrained refinement by Refmac [44] and Phenix.Refine [45] . Figures were drawn using either Coot [43] or PyMol [46] . For each structure, 284 amino acids of the native protein are visible in the molecule. Residues R26 to V40 and R184 to E194 could be fitted, but display higher flexibility as evidenced by less well-defined electron density. The bound ligands are clearly defined in both structures and refine well. A summary of the data collection and refinement statistics is given in Table 3 . Ramachandran statistics are 97, 3.2 and 0.0 % for most favoured, additionally allowed and disallowed residues of ATP-PRT/TIH and 98, 1.4 and 1.1% for ATP-PRT/ l- His. Native ion-mobility mass spectrometry On the day of analysis, the buffer was exchanged to 100 mM ammonium acetate buffer (Fisher Scientific, Loughborough, UK) of specified pH, using micro Bio-Spin Chromatography columns (Micro Bio-Spin 6 Columns, Tris) following the instructions specified by the manufacturer. The desalting procedure was performed four to five times to achieve desired sample quality. pH of the buffer was adjusted with ammonia supplied by VWR International Ltd (UK). Solution pH readings were taken using a pH metre (Jenway 3305). High purity water was obtained from an Arium 611 water purification unit (Sartorius, Göttingen, Germany) fitted with a 0.2 µm filter. The IM-MS data were acquired on a Synapt G2S HDMS (Waters, Manchester, UK). Samples were ionized using nano-elecrospray ionization (nESI) method, where protein species were charged and transferred from solution into the gas phase. nESI capillaries were prepared in-house from thin-walled borosilicate capillaries (inner diameter 0.9 mm, outer diameter 1.2 mm, World Precision Instruments, Stevenage, UK) using a Flaming/Brown P-97 micropipette puller (Sutter Instrument Company, Novato, CA, USA). These were then filled with sample using micro-loading tips (Eppendorf, Hamburg, Germany). A positive voltage was applied to the solution via 0.125 mm platinum wire (Goodfellow Cambridge Ltd., Huntingdon, UK) inserted into the capillary. Gentle conditions were applied to preserve the native-like structure: capillary voltage 1.6 kV, sampling cone 99 V, source temperature 20 °C, trap collision energy 5.6 V, and transfer collision energy 2 V. The pressure of the backing region was 8.3 mbar. For IM-MS, the helium cell and the IMS gas flows were 180 and 90 ml min −1 , respectively, the IMS wave velocity was 617 m s −1 , and the IMS wave height was 40 V. Nitrogen was the carrier gas. Data were acquired and processed with MassLynx software (Waters, Manchester, UK). Steady-state data analysis Steady-state data were fitted using the nonlinear, least-squares, curve-fitting programs of Sigma-Plot for Windows, version 11.0. Individual saturation curves were fit to Eq. 1 
    v = VS/( S + K)
 (1) where V is the maximal velocity, S is the substrate concentration, and K is the Michaelis constant for the substrate ( K m ). Inhibition data obtained under saturating concentrations of substrates and metals, and variable concentration of l- His, were fit to Eq. 2 
    v = v_0/[ 1 + ( I/IC_50)^n_H]
 (2) where v 0 is the uninhibited velocity, I is the l- His concentration, IC 50 is the concentration of l- His necessary to give 50% inhibition and n H is the Hill number. Activation data obtained under saturating concentrations of substrates and metals and variable concentration of TIH were fit to Eq. 3 [48] , [49] 
    v = v_0 + {[ (v_amax - v_0)×A^n_H]/[ AC_50^n_H + A^n_H]}
 (3) where v amax is the maximal velocity at maximum activation, A is the concentration of the activator TIH and AC 50 is the concentration of TIH necessary to increase the velocity by 50%. Activation data showing linear, non-essential activation pattern in a double-reciprocal plot were fit to Eq. 4 [38] , [39] 
    v = VS/{K[ ( 1 + A/K_A)/( 1 + β A/αK_A)] + S[ ( 1 + A/αK_A)/( 1 + β A/αK_A)]}
 (4) where K A is the activator dissociation constant, α is the constant that denotes the modification of the substrate and activator dissociation constants in the presence of each other and β is the constant of the modification of the catalytic constant. Inhibition data showing linear, uncompetitive patterns in double-reciprocal plots were fit to Eq. 5 
    v = VS/[ K + S( 1 + I/K_i)]
 (5) where K i is the dissociation constant for the enzyme-inhibitor complex. Inhibition data showing linear, noncompetitive patterns in double-reciprocal plots were fit to Eq. 6 
    v = VS/[ K( 1 + I/K_i) + S( 1 + I/K_i)]
 (6) Tertiary replots of the slopes and intercepts against activator concentration were fit to Eq. 7 [50] 
    Slope/Intercept = [ y_0 + y_∞( A/K_A)]/[ 1 + ( A/K_A)]
 (7) where y 0 is the value of slope or intercept in the absence of activator and y ∞ is the value of slope or intercept in the presence of infinite concentration of activator. Data availability The atomic coordinates and the structure factors for M. tuberculosis ATP-PRT in complex with l- His and TIH have been deposited into the Protein Data Bank under the accession codes 5LHU and 5LHT. The UniProt accession codes P9WMN1 and P9WI55 for M. tuberculosis ATP-PRT and PPiase, respectively were used in this study. All other data are available from the corresponding author on reasonable request.